Enhancing far-field thermal emission with thermal extraction The control of thermal radiation is of great current importance for applications such as energy conversions and radiative cooling. Here we show theoretically that the thermal emission of a finite-size blackbody emitter can be enhanced in a thermal extraction scheme, where one places the emitter in optical contact with an extraction device consisting of a transparent object, as long as both the emitter and the extraction device have an internal density of state higher than vacuum, and the extraction device has an area larger than the emitter and moreover has a geometry that enables light extraction. As an experimental demonstration of the thermal extraction scheme, we observe a four-fold enhancement of the far-field thermal emission of a carbon-black emitter having an emissivity of 0.85. An idealized macroscopic blackbody emitter of an area S at a temperature T , in direct contact with free space ( Fig. 1a ), has a total emission to far-field vacuum of σT 4 S , where σ is the Stefan–Boltzmann constant, as prescribed by the well-known Stefan–Boltzman law. Any actual macroscopic thermal body cannot emit more thermal radiation than a blackbody. The Stefan–Boltzman law provides an important theoretical foundation for much of the recent works aiming to design nanophotonic structures in order to tailor the spatial and spectral properties of far-field thermal emission [1] , [2] , [3] , [4] , [5] , [6] , [7] , [8] , [9] , [10] , [11] , [12] , [13] , [14] , [15] , [16] , [17] , [18] , [19] . 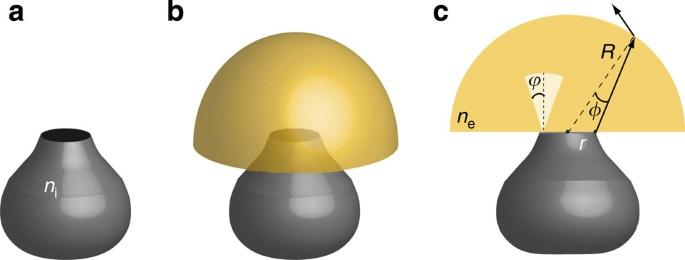Figure 1: Schematic of thermal extraction. (a) Emitter formed by an open area (black surface) of an absorptive cavity. The cavity can be filled with transparent dielectric of refractive indexni. (b) Thermal extraction using a hemispherical dome placed at the opening of the cavity. The dome is transparent and does not emit or absorb any thermal radiations, and has a refractive indexne. (c) Cross-section showing emission cone (white) of the thermal radiation inside the dome. Figure 1: Schematic of thermal extraction. ( a ) Emitter formed by an open area (black surface) of an absorptive cavity. The cavity can be filled with transparent dielectric of refractive index n i . ( b ) Thermal extraction using a hemispherical dome placed at the opening of the cavity. The dome is transparent and does not emit or absorb any thermal radiations, and has a refractive index n e . ( c ) Cross-section showing emission cone (white) of the thermal radiation inside the dome. Full size image In this Letter, in contrast to the standard geometry that Stefan–Boltzman law is applied as shown in Fig. 1a , we consider an alternative geometry, as shown in Fig. 1b , where the emitter is instead in contact with a thermal extraction device such as a hemispherical dome that is transparent. In this case, we show both theoretically and experimentally that, under proper conditions, the emission to far-field vacuum can exceed σT 4 S , in spite of the fact that the thermal extraction device itself is completely transparent and does not emit any thermal radiation. We emphasize that our results do not violate the Stefan–Boltzman law, as the physical area of the thermal extraction device is larger than the emitter itself. In this sense our results are fundamentally different from near-field thermal transfer experiments where Stefan–Boltzman law does not apply [20] , [21] , [22] , [23] , [24] , [25] . Our finding here is consistent with known physics of radiometry including the consideration of optical etendue conservation [26] . Thermal extraction also shares similar physical principles with light extraction used in light emitting diode [27] , [28] , and solid immersion lenses used for resolution enhancement [29] . Analysis of thermal extraction with a cavity blackbody model To illustrate our concepts we start by briefly reviewing the cavity model description of a blackbody emitter, which consists of a small opening on a cavity shown in Fig. 1a . The idea is equally applicable to other implementations of blackbodies. The cavity has vacuum immediately outside. The opening has an area S . The inner sidewall of the cavity is made of diffusive reflector that also absorbs light. The opening area is completely dark with emissivity of unity: any light entering through the open area bounces many times and eventually gets absorbed by the sidewall. The cavity is maintained at temperature T . We further assume the cavity is filled with transparent dielectric medium that has a refractive index n i . (Below, we refer the cavity with n i =1 as an ‘empty cavity’, and with n i >1 as a ‘filled cavity)’. Perfect antireflection is assumed at all interfaces. In this case, it is well known [30] that independent of the value of refractive index n i , the cavity always has the same external thermal emission characteristics with the same total emitted power σT 4 S to far-field vacuum. Inside the cavity, the internal thermal radiation intensity scales as n i 2 as it is dependent on the electromagnetic density of states. However, when n i >1, total internal reflection, occurring at the interface between the medium inside the cavity and vacuum outside, prevents significant portion of the internal electromagnetic modes from coupling to vacuum. The resulting thermal emission to the far-field thus has the same profile independent of internal radiation intensity. As the main result of our paper, we now demonstrate that for the emitter in Fig. 1a , one can enhance its thermal emission by placing a hemispherical dome with refractive index n e covering the entrance of the cavity, as shown in Fig. 1b . The dome is in close contact with the open area of the cavity. Here the dome plays the role of a thermal extraction device that enables all modes inside the cavity to escape into vacuum. Importantly, the dome itself is assumed to be transparent, so that it does not emit or absorb any thermal radiation. To calculate the thermal emission from the geometry shown in Fig. 1b , we follow a ray tracing procedure. For simplicity, we assume that the opening of the cavity has a circular shape of radius r and the dome has a radius R . We further assume R ≥ n e r , which is sufficient to ensure that any light ray originated from the open area S , when it reaches the top surface of the dome, has an incident angle less than the total internal reflection angle φ ≤sin −1 (1/ n e ) ( Fig. 1c , solid arrows), and, therefore, can escape to far-field vacuum (see Supplementary Fig. S1 ). Here again we assume perfect antireflection at the dome surface. The emission from the cavity forms a light cone in the dome. Half apex angle of the light cone is given by To obtain the total emission power, we integrate thermal radiation within the light cone, As all lights in the dome can escape without total internal reflection, Equation (2) is the total thermal radiation to far-field vacuum. 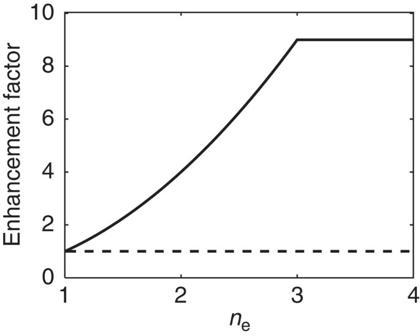Figure 2: Enhancement of far-field radiation power as a function of the refractive index of the domene. Enhancement is compared withσT4SThe structure is for enhancement is shown inFig. 1b. Solid line: Filled cavity withni=3. Dashed line: Empty cavity withni=1. Figure 2 shows the thermal radiation as a function of the refractive index of the dome n e . The total radiation power from an empty cavity (dashed line in Fig. 2 ) does not change as a function of n e , while the power from the filled cavity (solid line in Fig. 2 ) increases as n e increases until n e = n i . With the assistance of the thermal extraction, the filled cavity can emit up to n i 2 S σ T 4 to far-field vacuum, n i 2 times of power without thermal extraction. Figure 2: Enhancement of far-field radiation power as a function of the refractive index of the dome n e . Enhancement is compared with σT 4 S The structure is for enhancement is shown in Fig. 1b . Solid line: Filled cavity with n i =3. Dashed line: Empty cavity with n i =1. Full size image It is well-known that when in contact with a transparent medium with index higher than vacuum, an ideal blackbody emits more thermal radiation into the transparent medium as compared with the same blackbody to vacuum [25] . Our use of hemispherical dome exploits this fact, and also ensures that all radiation into the high-index dome can escape to vacuum, leading to enhanced far-field thermal radiation. Moreover, our theory above indicates that the internal density of state of the blackbody is in fact important to achieve such emission enhancement. As can be seen in Fig. 2 , the internal density of state of the thermal body must be higher than that of the extraction device in order to achieve the maximum effect of enhanced thermal emission. The distribution of thermal radiation on the surface of the dome can be calculated with a schematic shown in Fig. 3a . 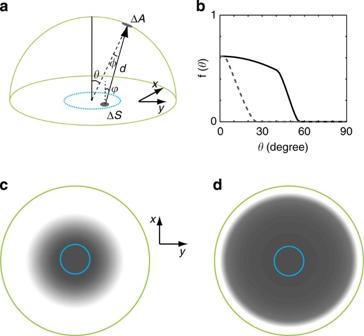Figure 3: Distribution of thermal radiation on the surface of the extraction dome. (a) Schematic of the calculation. Solid arrow indicates radiation that is emitted from a small area ΔSon the cavity opening and is received by a small area ΔAon the surface of the dome. (b) Distribution of the radiation power on the surface of the dome as a function of the polar angleθ. Dashed and solid lines are for the cases with empty and filled cavities, respectively. (c,d) The distribution of the radiation power, plotted on the hemisphere of the dome, for the case of empty (c) and filled (d) cavity. The blue circle indicates the emitter area, that is, the opening area of the cavity. The green circle is the boundary of the dome. Darker region indicates higher emission and the white region has zero emission. For a small area Δ A on the surface of the dome, the thermal radiation power it receives from the cavity is Figure 3: Distribution of thermal radiation on the surface of the extraction dome. ( a ) Schematic of the calculation. Solid arrow indicates radiation that is emitted from a small area Δ S on the cavity opening and is received by a small area Δ A on the surface of the dome. ( b ) Distribution of the radiation power on the surface of the dome as a function of the polar angle θ . Dashed and solid lines are for the cases with empty and filled cavities, respectively. ( c , d ) The distribution of the radiation power, plotted on the hemisphere of the dome, for the case of empty ( c ) and filled ( d ) cavity. The blue circle indicates the emitter area, that is, the opening area of the cavity. The green circle is the boundary of the dome. Darker region indicates higher emission and the white region has zero emission. Full size image The definitions of the geometric parameters in Eq. (3) are provided in Fig. 3a and φ i is the maximum apex angle as defined in Eq. (1). All radiation that the area Δ A receives can escape the dome. As a dimensionless quantity, we define a normalized power distribution to describe the power distribution on the surface of the dome. Owing to rotational symmetry, f depends only on the polar angle θ . As one specific numerical example, we calculate a case where n e =4. We choose the dome radius R =5 r to satisfy the condition R ≥ n e r . f ( θ ) is numerically evaluated using Equation (3) and is shown in Fig. 3b for both empty cavity ( n i =1) ( Fig. 3c ), and filled cavity ( n i =3) ( Fig. 3d ). For both cases, f ( θ ) never exceeds unity. This is expected from the Stefan–Boltzman law: as the dome is in direct contact with vacuum outside, the emission from every surface element of the dome cannot exceed that of a surface element on a blackbody with the same area. We see that f ( θ ) maximizes at normal direction θ =0, as this area is directly above the opening the cavity. f ( θ ) decreases as θ increases and eventually vanishes for large θ , as at large θ the corresponding area lies outside the emission cone of cavity. However, the emission profile of the filled cavity expands to a much wider angular range than that of the empty cavity ( Fig. 4c ). When thermal extraction occurs, as for example for the case here of the filled cavity, the entire dome appears bright. Therefore, the use of the transparent dome allows one to enlarge the actual emission area beyond the physical area of the emitter itself and, therefore, enhances the thermal emission. 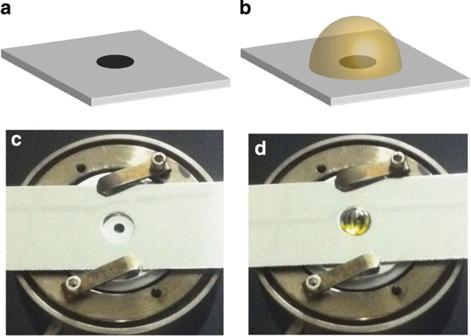Figure 4: Schematic and actual experimental structure for demonstration of thermal extraction. (a,c) Emission source made of carbon dot is coated on an aluminium plate placed on a temperature-controlled heater. (b,d) Thermal extraction device made of ZnSe hemisphere is placed in close contact with carbon dot. Figure 4: Schematic and actual experimental structure for demonstration of thermal extraction. ( a , c ) Emission source made of carbon dot is coated on an aluminium plate placed on a temperature-controlled heater. ( b , d ) Thermal extraction device made of ZnSe hemisphere is placed in close contact with carbon dot. Full size image Experimental demonstration of thermal extraction Based on the theoretical analysis above, we now experimentally demonstrate the use of thermal extraction to enhance thermal emission of a carbon-black thermal body. It has a refractive index around 2.3 and an emissivity around 0.85 in the near to mid-infrared regime. A circular carbon dot is coated on a polished Al sample holder, which provides a low emission background. The dot has a radius r =1.025 mm with an area of 3.3 mm 2 ( Fig. 4a ). For the thermal extraction device, we use a hemispherical dome made from ZnSe, a transparent material with negligible thermal emission in the near to mid-infrared (IR) region. The hemisphere has a diameter of 6 mm and refractive index 2.4 ( Fig. 4b ). It satisfies the condition R ≥ n e r , which ensures that light entering into the hemisphere from the thermal emitter is not trapped by the total internal reflection at the dome interface. The aluminium sample holder is placed on a temperature-controlled heater ( Fig. 4c ). The entire heater is placed in a vacuum chamber (~10 −6 torr) to avoid oxidation of ZnSe and to maintain thermal stability. The source is observed through a CaF 2 window on the vacuum chamber. The thermal emission is collected by a parabolic mirror and sent through an aperture to a Fourier transform infrared (FTIR) spectrometer. The use of the aperture allows us to collect emission from only a small area on the sample holder. For each measurement, we centre the collection area on the source by adjusting the position of the aperture until maximum reading is reached. To measure the angular emission, the heater stage can be rotated inside the vacuum chamber. For calibration purposes, a blackbody simulator (Infrared System Development Corporation 564/301 and IR-301 Blackbody controller) is also measured using the same optical set-up. By comparing to such calibration measurement, we can, therefore, obtain the absolute power emission from our thermal emitters ( Supplementary Fig. S2 ). The sample is maintained at 553 K. Temperature consistency is confirmed by both the thermal controller and the emission spectra ( Supplementary Fig. S3 ). Background emission from the Al sample holder is also characterized and has been subtracted out in the data shown below ( Supplementary Fig. S4 ). 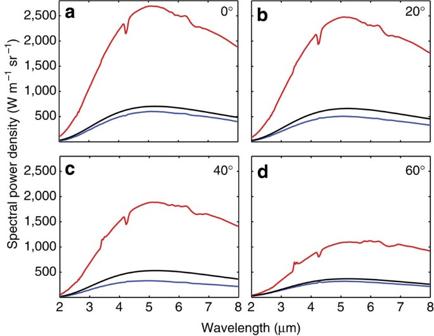Figure 5: Emitted power spectra measured at 553 K for different collection angles. Red and blue lines are for the carbon dot with and without the hemispherical dome, respectively. Black lines are emission power from an ideal blackbody of the same area as the carbon dot at the same temperature. The ripples in the curves are caused by atmosphere absorption. (a), (b), (c), and (d) are measured at 0, 20, 40, and 60 degrees, respectively. Figure 5 shows the emission spectra of the structures at various angles. The emission peaks at 5.25 μm wavelength, as expected for a near-black emitter at a temperature of 553 K. The spectral density from an ideal blackbody of the same size as the carbon-black dot is plotted as reference (black lines). As expected, the bare carbon dot (blue lines) emits less than the ideal blackbody, with an emissivity of 0.85 in the normal direction. In the presence of the dome, the emitted power in the normal direction from the same carbon-black dot is enhanced by 4.46-fold, representing a 3.79-fold enhancement over the emission by an ideal blackbody with the same area as the carbon-black dot ( Fig. 5a ). Similar enhancement is observed for off normal directions as well ( Fig. 5b–d ). The enhanced emission is purely from the extraction of carbon’s internal thermal energy, not from the ZnSe hemisphere. To verify this, a reference sample with the ZnSe hemisphere but without the carbon dot is measured, and it shows negligible emission ( Supplementary Fig. S4 ). Figure 5: Emitted power spectra measured at 553 K for different collection angles. Red and blue lines are for the carbon dot with and without the hemispherical dome, respectively. Black lines are emission power from an ideal blackbody of the same area as the carbon dot at the same temperature. The ripples in the curves are caused by atmosphere absorption. ( a ), ( b ), ( c ), and ( d ) are measured at 0, 20, 40, and 60 degrees, respectively. 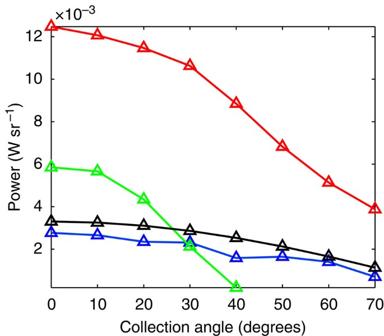Figure 6: Experimentally measured emission power from the carbon dot as a function of angle. Red and blue is for with and without the ZnSe hemispherical dome in optical contact, respectively. Green is for the case where the flat surface of the dome is separated from the carbon dot by 30 μm. Triangles are measured data points. The black line is the emission power from an ideal blackbody with the same area as the carbon dot. Full size image Figure 6 shows the angular emission, as obtained by integrating the spectral density over the wavelength range of 2–8 μm. For all angles, the presence of the dome results in enhanced emission ( Fig. 6 , red curve), as compared with both the carbon-black dot without the dome ( Fig. 6 , blue curve) and an ideal thermal body ( Fig. 6 , black curve) of the same area. The total thermal emission is obtained by integrating over all angles and all wavelengths in the range of 2–8 μm. The total emission is 10.4 mW for the ideal thermal body, 7.6 mW for the bare carbon dot and 31.3 mW for the carbon dot with the dome. Figure 6: Experimentally measured emission power from the carbon dot as a function of angle. Red and blue is for with and without the ZnSe hemispherical dome in optical contact, respectively. Green is for the case where the flat surface of the dome is separated from the carbon dot by 30 μm. Triangles are measured data points. The black line is the emission power from an ideal blackbody with the same area as the carbon dot. Full size image The hemispherical dome we use here is a focusing lens. However, the thermal extraction effect is fundamentally different from the far-field focusing effect of the lens. To achieve thermal extraction, we require that all internal states of the emitters can couple into the modes inside the dome. Thus the emitter and the dome must be in optical contact, that is, the distance between the emitter and the flat surface of the dome must be significantly smaller than the thermal wavelength. Preventing the optical contact between the emitter and the dome should eliminate the thermal extraction effect. As a demonstration, we conduct a comparison experiment where the dome is lifted away from the carbon dot by 30 μm, a distance that is large enough to prevent photon tunnelling between the emitter and the dome, and small enough to preserve all other geometrical optical lens effects ( Fig. 7c ). The resulting emission power is shown as green line in Fig. 6 . In the normal direction, due to the focusing effect of the hemispherical dome, the emission is higher than that that of bare carbon dot, but it quickly diminishes at large angles with negligible emission beyond 40°. Therefore, the geometrical optical effect of ZnSe hemispherical dome can only redistribute the thermal emission but does not enhance the total emission. The total emitted power is only 4.1 mW, below that from the ideal thermal body with the same area at the same temperature. 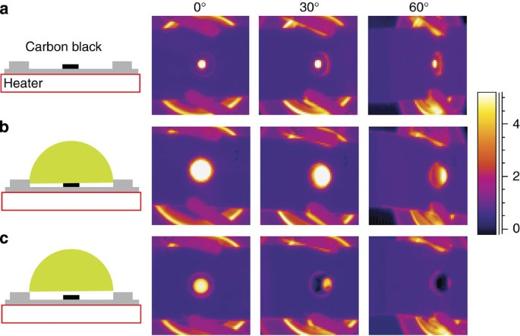Figure 7: Infrared images of the thermal sources maintained at a temperature of 553 K. Images are taken at 0, 30 and 60°. All images have the same colour scale. Values on the colour scale bar are linearly proportional to the photon counts of detectors in the camera. In all images, the most outer bright regions are the heater surface beneath the Al sample holder. (a) Bare carbon dot. The Al plate has a holder for the hemisphere, the edge of which is visible due to its slightly higher emissivity. (b) The carbon dot is in optical contact with ZnSe. Notice that the entire dome lights up at the normal direction and significant emission even at 60° angle, demonstrating thermal extraction. (c) ZnSe hemisphere is spaced away from carbon dot by 30 μm, a distance sufficient to prevent thermal extraction. In this case, ZnSe hemisphere only redistributes emission among different directions. Figure 7: Infrared images of the thermal sources maintained at a temperature of 553 K. Images are taken at 0, 30 and 60°. All images have the same colour scale. Values on the colour scale bar are linearly proportional to the photon counts of detectors in the camera. In all images, the most outer bright regions are the heater surface beneath the Al sample holder. ( a ) Bare carbon dot. The Al plate has a holder for the hemisphere, the edge of which is visible due to its slightly higher emissivity. ( b ) The carbon dot is in optical contact with ZnSe. Notice that the entire dome lights up at the normal direction and significant emission even at 60° angle, demonstrating thermal extraction. ( c ) ZnSe hemisphere is spaced away from carbon dot by 30 μm, a distance sufficient to prevent thermal extraction. In this case, ZnSe hemisphere only redistributes emission among different directions. Full size image As we have seen in the analysis of Fig. 3 , the thermal extraction effect is directly correlated with a broadening of angular distribution of photons on the dome surface. When thermal extraction occurs, the apparent emitting area thus should appear larger from all viewing angles. To demonstrate this, we directly visualize the emitters with an IR camera (FLIR System Inc. SC4000, spectral range 3–5 μm) ( Fig. 7 ). We compare three cases: the bare carbon dot, the carbon dot in optical contact with the ZnSe dome and the carbon dot separated from the ZnSe dome by 30 μm. For all three cases, the emitting sources are the same, but as we have already seen in Figs 5 and 6 , the emitted powers are drastically different. Such differences can be directly visualized with the camera. The bare carbon dot has an emission profile that is approximately Lambertian. The apparent emitting area reduces with increasing angle ( Fig. 7a ). When the carbon dot is in optical contact with the hemispherical lens ( Fig. 7b ), the effect of thermal extraction produces much larger apparent emitting area for all viewing angles. This agrees with the angular distribution calculation shown in Fig. 3 . Figure 7c shows the case where the ZnSe hemisphere is spaced away from the carbon dot. At normal direction, the apparent emitting area is larger as compared with that of the bare dot. But the apparent emitting area decreases very rapidly with angles. At large angles, the apparent emitter area is smaller compared with the case of the bare dot. This again is consistent with the results of Fig. 6 , showing that thermal extraction is fundamentally different from a focusing effect. We have illustrated the concept of thermal extraction with the example of a high-index hemispherical dome. In general, thermal extraction can be accomplished with other geometries as well. Here we comment on the general requirement of the thermal extraction device: Firstly, the thermal extraction needs to be in optical contact with the emitter, that is, the distance between the emitter and the extraction device needs to be smaller compared with the evanescent length scale determined by the thermal wavelength λ T = ħc / k B T . This is to ensure that all internal states in the emitter can couple to modes in the extraction device. We note, however, the thermal extraction device needs not be in physical contact with the emitter. This could be useful in practice when it is advantageous to prevent thermal conduction between the extraction device and the emitter. Secondly, from a thermodynamics point of view, the thermal extraction device needs to provide enough radiation channels [31] over the area of the emitter to ensure that all internal modes of the emitter can out-couple. A simple way to accomplish this is to choose the extraction device such that its density of states is larger than that of the emitter. The size of the extraction device also needs to be sufficiently large, such that the vacuum region immediately outside the extraction device has sufficient number of radiation channels to accommodate all the thermal emission. Both of these considerations are incorporated in our choice of parameters for the hemispherical dome. On the other hand, based upon these considerations, one can envision a wide variety of nanophotonic structures that may satisfy these thermodynamic considerations. For example, structured materials, for example, photonic crystal and metamaterial, can be engineered to have extremely high channel density. Their dispersion relations can also be tailored such that extracted radiations can be guided to vacuum interfaces where enough channels in vacuum are available to accommodate the radiation. Finally, in the extraction device those optical modes that receive radiation from the emitter need to be accessible to far-field vacuum. This places a constraint on the geometry of the extraction device. For example, a transparent high-index slab with flat surface does not provide thermal extraction. Even though more radiation can enter the slab, those outside the escape cone defined by sin −1 (1/ n e ) cannot escape to far-field vacuum due to total internal reflection. As a result, the total far-field emission remains the same as SσT 4 . This particular requirement on making internal optical states accessible to far-field shares the same spirit of the requirement on light trapping in solar cells [31] , [32] , [33] . Many light trapping structures, for example, roughened slab, irregular polygon and nanostructured interface can be directly used for thermal extraction. The demonstration of thermal extraction here opens possibilities for a number of applications. For example, there is a strong effort seeking to miniaturize the active emitting region of a thermal source, as with a smaller active region [18] , it takes less power to drive the active region to a prescribed temperature. However, at a constant temperature miniaturization of the active region typically comes with the price of reduction in emitted power. Here we show that it is actually possible to decouple the area of the active emitter and its emitted power, which may potentially lead to a better thermal emitter with higher power efficiency. Thermal extraction also indicates the possibility of enhancing thermal transport in the far-field for efficient radiative cooling and heating [34] . Total internal reflection condition in hemispherical domes We consider the geometry shown in Supplementary Fig. S1 , and derive the condition that allows emission from the source area to escape from the dome without total internal reflection. The emitting area has a radius r . The dome has a radius R . At the surface of the dome, the incident angle of the ray is φ . Using the sine rule, we have sin( φ )= r sin( θ )/ R . As a worst-case scenario, we assume a maximum emission cone from the source to the dome, that is, the maximum value for θ is 90°. To prevent the total internal reflection, we require that sin( φ )≤1/ n e . With these considerations, we therefore have R ≥ rn e . Transfer function of the measurement system The raw data measured by the FTIR system is in an arbitrary linear unit. Supplementary Fig. S2 shows the raw data measured for the bare carbon dot, and the carbon dot in optical contact with the ZnSe dome, both at a temperature of 553 K. To convert this arbitrary unit to power measurement, we need to know the transfer function of the system. We obtain the transfer function by calibrating the system to a known blackbody emitter simulator (Infrared System Development Corporation 564/301 and IR-301 Blackbody controller). The blackbody simulator consists of a cone cavity with black absorptive inner surface. The open area of the cone has emissivity over 0.99. The emission is collected by the same optical configuration. The collection area is controlled by the aperture size. By assuming the known emitter as an ideal blackbody and thus having a standard Planck’s law emission, we can obtain the transfer function of the system shown in Supplementary Fig. S3 . The transfer function converts the measured FTIR signal to absolute power emission. Determination of temperature The samples are maintained at the same temperature for measurement. The heater controller is set to be the same temperature for all measurement. The samples are placed on the heater surface in vacuum, and thus isolated from heat transfer by conduction and convection. Measurements are performed 45 min after the set temperature is reached to help the sample reach steady state. The temperate consistency for different measurement is confirmed by the lineshapes of the emission. Supplementary Fig. S3 shows the normalized lineshapes for the emission measured for the bare carbon dot (blue), and the carbon dot in optical contact with the dome (red). These lineshapes overlap very well, showing that they are at the same temperature. We match the emission lineshapes of the samples to those of a reference blackbody simulator (Infrared System Development Corporation 564/301 ) to obtain the sample surface temperature. This is accurate as the carbon-black’s emissivity has little wavelength dependency in the measured spectral range. The reference blackbody emitter’s temperature is maintained by Infrared System Development Corporation IR-301 Blackbody controller. Spectra of the reference blackbody are measured from 533 to 573 K ( Supplementary Fig. S3 dashed lines). The 553 K lineshape shows the best match with the sample spectra ( Supplementary Fig. S3a ), while 533 and 573 K show significant deviation ( Supplementary Fig. S3b,c ). The sample temperature is determined to be 553±10 K. Background emission The aluminium sample holder has small but finite emission. In this section, we describe the experiments to determine the background emission by the sample holder including the ZnSe hemisphere. We also show that the ZnSe hemisphere by itself emits very little thermal radiation. First, the sample holder without carbon dot is measured ( Supplementary Fig. S4a ). Its emission is shown by Supplementary Fig. S4c dashed line. The collection area is slightly larger than the centre circular aperture shown in Supplementary Fig. S4a . The collection area includes a circular edge, which is used later on to fix the ZnSe hemisphere. Then, carbon dot is coated on the Al sample holder ( Supplementary Fig. S4b ). Despite its small area compared with the collection area, the carbon dot dominates the emission as compared with the background emission from the aluminium sample holder ( Supplementary Fig. S4c solid line). The emission shown in the main text is obtained by subtracting out the background emission. Similarly, measurements are performed for the ZnSe hemisphere without the carbon dot ( Supplementary Fig. S4d ). ZnSe does not have significant thermal emission, as can be seen by comparing the dashed lines in Supplementary Fig. S4c,f . The enhanced thermal emission in Supplementary Fig. S4f , in the presence of the carbon dot, is purely from extracting the internal thermal radiation energy from the carbon dot. Infrared spectroradiometer The measurement of spectral radiance from the heated sample is performed with a custom built vacuum emissometer ( Supplementary Fig. S5a ). The sample holder is based on a 1′′ diameter high-temperature heater (HeatWave Labs Model 104863-02) in an ultrahigh vacuum chamber ( Supplementary Fig. S5b ). Samples are mounted on the heater. A feed through mechanism allows rotation of the heater in vacuum, in order to measure the angular dependence of the spectral radiance. The axis of rotation is in the plane on which the sample is mounted, thus minimizing sample displacement during rotation. The directional spectral radiance emitted by samples is observed outside the vacuum chamber through a CaF 2 window. External imaging and collimating optics are used to guide the spectral radiance into the entry port of FTIR spectrometer ( Supplementary Fig. S5a ) (FTIR: Nicolet 6700 with CaF 2 beam splitter and deuterated triglycine sulphate detector with KBr window). The external optical set-up consists of a collection and a collimation system. A gold-coated 90° off-axis parabolic mirror with focal length f =152.4 mm and diameter D =50.88 mm (Edmund Optics NT47-110) are used to collect the emitted radiation. This mirror images the sample plane onto a tunable aperture. The aperture is tuned in both diameter and position to select the size and the location of the collection area on the sample. A second gold-coated 90° off-axis parabolic mirror with focal length f =203.2 mm and diameter D =38.1 mm (Newport 50332AU) is used to collimate the light from the aperture into the entry port of the FTIR spectrometer. Infrared images We use an infrared camera based on an InSb photodiode array image sensor with 320 × 256 pixels. The specified spectral range is 3.0–5.0 μm. Images are read out as raw data, which are proportional to the received number of photons within the spectral range of the camera ( Supplementary Fig. S6 ). Pixel-to-pixel responsivity variations are negligible for the purposes of this work. The camera views the sample through the CaF 2 window on the vacuum chamber via a plane gold mirror with high reflectance. A 50-mm focal length f/2.5 lens was used. The sample holder allows observation of the emission source for angles out to about 70° (with some obscuration occurring at larger angles). Images below show the progression of the source emission with increasing off-axis angle. The artificial colour scale is the same in all images. Quantitative analysis based on infrared images The apparent emission area is enhanced by the presence of the dome. The enhancement is dependent on the viewing angles and also in particular, the distance between the dome and the carbon dot. These images also allow us to perform a quantitative analysis on the emission power. The analysis of the images relies on assumptions to a larger extent than for the FTIR measurement. Notably, the camera images do not allow a check on the temperature, which is provided by the FTIR through the lineshape. Also, the camera does not measure the power directly, but rather the flux of photons within its relatively narrow spectral range. On the other hand, the camera provides a direct visualization of the thermal extraction and expansion of the apparent emission area due to the conservation of optical etendue. The camera images have been analysed as follows: The camera is calibrated for a temperature of 280 °C using the blackbody source. In the images of the sample, pixel values are first divided by the mean pixel reading in the 280 °C blackbody calibration. To represent the result on a scale comparable to Fig. 6 in the main paper, pixel values were multiplied by the intensity of an ideal blackbody at 280 °C with area equal to the pixel area at the sample. The image region containing the source was segmented out by thresholding the image at 2/3 of the peak pixel intensity above background. The pixel values in this region were added together, giving the intensity (W/sr) of the source in the chosen viewing direction. The result of image analysis is shown in Supplementary Fig. S7 . The overall trend is consistent with Fig. 6 in the main paper. How to cite this article: Yu, Z. et al . Enhancing far-field thermal emission with thermal extraction. Nat. Commun. 4:1730 doi: 10.1038/ncomms2765 (2013).